RETRACTED ARTICLE: Senescence impairs direct conversion of human somatic cells to neurons Recent reports have shown that fibroblasts can be converted to neurons by forced expression of transcription factors. However, the mechanisms underlying this conversion remain unclear. Here, we show that the efficiency of neuronal conversion of embryonic human fibroblasts aged in culture is lower than that in cells in early culture stages. Moreover, depletion of p16 Ink4a and p19 Arf involved in the activation of cellular senescence is sufficient to convert human fibroblast and epithelial cells into neurons. The induced neurons express neuron-specific proteins, generate action potentials and neurotransmitter receptor-mediated currents. Genome-wide transcriptional analysis shows that the induced neurons have a profile different from fibroblasts and similar to that of control neurons induced by established methods. We further noted that expression of p53 blocks the neuronal conversion, whereas expression of human telomerase reverse transcriptase (hTERT) induces it. Our results indicate that overcoming senescence is a crucial step for neuronal conversion of somatic cells. Somatic cells can be reprogrammed to form embryonic stem cell-like induced pluripotent stem (iPS) cells by forced expression of a set of transcription factors [1] , indicating that terminally differentiated cells can be induced to undergo cell fate change. Recently direct conversion from fibroblasts to neurons bypassing the pluripotent state has been demonstrated [2] , [3] , [4] , [5] , [6] , [7] , [8] , [9] , [10] , [11] , [12] , [13] , [14] . However, the conversion takes a few months with low percentages of success, likely because of a poor understanding of the underlying mechanisms and the existence of barriers limiting its efficiency. Cellular senescence has been shown to inhibit reprogramming of fibroblasts to iPS cells [15] , [16] , which raised the possibility that they might suppress fibroblast conversion to neurons. Cellular senescence is often the consequence of culture-induced upregulation of p16 Ink4a and p19 Arf , as well as activation of p53 (refs 17 , 18 , 19 , 20 , 21 ), implicating that these genes might block fibroblast–neuron conversion. Here, we investigate whether p16 and p19 controls direct conversion of fibroblasts to neuronal cells. We find that depletion of p16 or p19 alone can efficiently convert human fibroblasts into functional neurons. Overexpression of human telomerase reverse transcriptase (hTERT) in primary human fibroblasts, which can prevent cellular senescence and lead to immortalization, also induces neuron formation. Thus, these data indicate that blocking cellular senescence pathways eliminates a roadblock during fibroblast–neuron conversion. Depletion of p16 or p19 induces fibroblasts into neurons Lentiviral constructs expressing short hairpin RNA against p16 and/or p19 were transfected to human embryonic lung-derived fibroblasts (IMR90) cells ( Fig. 1a ). Western blot analysis showed significant decreases of p16 and p19 expression by shRNAs in IMR90 cells ( Fig. 1b ). We cultured IMR90 fibroblasts with the expression of p16, p16/p19 or p19 shRNA in a defined neuronal induction medium for neuron induction ( Fig. 1a and see Methods section). In only 2–3 days, we observed bipolar neuron-like cells. In 7 days, cells with more mature neuronal morphology that expressed both TUJ1 (a neuronal marker) and MAP2 (a marker of post-mitotic neurons) were present ( Fig. 1c ). In 3–4 weeks, 60–85% of fibroblasts were transdifferentiated into induced neuronal (iN) cells ( Fig. 1d ; iN purity, based on MAP2+ cells). We calculated the iN yield as the percentage of MAP2+ cells in relation to the initial number of plated fibroblasts. At 3 weeks after induction, we obtained yields of 55±15%, 34±11% and 58±12% for shp16, shp19 and shp16/19, respectively ( Fig. 1e ). In contrast, after 4 weeks in neuronal medium, control IMR90 cells (untreated and empty vector) kept fibroblast morphology with negative staining of MAP2 ( Fig. 1c,d ; Supplementary Fig. 1 ). These results suggest that p16–p19 deficiency led to direct conversion of human fibroblasts to neurons. To confirm the effect of p16–p19 knockdown on conversion of iN cells, we expressed shp16 and shp19 in a line of human fetal lung fibroblasts WI38 and adult dermal fibroblasts derived from a 46-year old healthy male donor. Expression of shp16–shp19 converted WI38 and adult dermal fibroblasts to iN cells three weeks after induction ( Fig. 2a–c ), whereas control cells still kept fibroblast morphology. Thus, transient inactivation of p16–p19 by shRNAs is sufficient to directly convert fibroblasts into neurons. To investigate whether p16–p19 has a general effect on human somatic cells, we also expressed shp16 and shp19 in primary human epithelia cells from bronchus/trachea tissues of a 34-year-old female donor. After induction for 3 weeks in a modified induction medium, about 15–20% epithelia cells were converted into neurons ( Fig. 2a–c ). iN cells were positive in the immunostaining of TUJ1 and MAP2, similar to iN cells from IMR90 cells. Thus, inactivation of p16–p19 is able to convert different somatic cells into neurons. 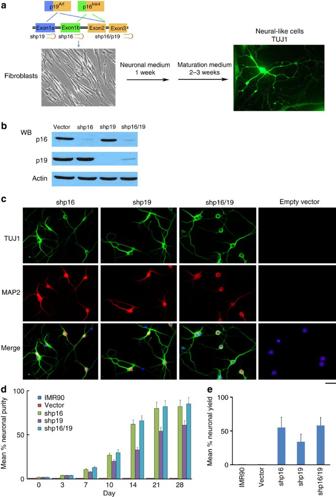Figure 1: Direct conversion of human fibroblasts into neuronal cells byp16andp19shRNAs. (a) Schematic drawing of the structure of theInk4a/Arflocus and the experimental strategy to derive induced neural cells. The images show the IMR90 fibroblast morphology and TUJ1-positive iN cells (shp16) with multiple neurites processing out of the cell body 4 weeks after induction. (b) Depletion ofp16, p19andp16/p19by shRNAs. Western blot analysis shows decrease of p16 and p19 expression by shRNAs in IMR90 cells. (c) Characterization of neuronal cells derived from shp16, shp19 and shp16/19 IMR90 cells. The images show the TUJ1- and MAP2- positive iN cells from shp16, shp19 and shp16/19 IMR90 fibroblasts 3 weeks after induction. Scale bar, 10 μm. (dande) Quantitative analysis of iN cells from IMR90 cells with or without expressing shp16, shp19 or empty vector after induction. Kinetic analysis of iN purity was counted by morphology, TUJ1- (early stage, before one week induction) and MAP2-positive (late stage, after 1 week induction) staining, and the numbers represent the percentage of iN cells at the time point of quantification (d). Neuronal yield was determined as the percentage of MAP2+ cells in relation to the initial number of plated fibroblasts at 3 week after induction (e). Quantitative data were mean±s.e.m. from at least three independent experiments. Figure 1: Direct conversion of human fibroblasts into neuronal cells by p16 and p19 shRNAs. ( a ) Schematic drawing of the structure of the Ink4a/Arf locus and the experimental strategy to derive induced neural cells. The images show the IMR90 fibroblast morphology and TUJ1-positive iN cells (shp16) with multiple neurites processing out of the cell body 4 weeks after induction. ( b ) Depletion of p16, p19 and p16/p19 by shRNAs. Western blot analysis shows decrease of p16 and p19 expression by shRNAs in IMR90 cells. ( c ) Characterization of neuronal cells derived from shp16, shp19 and shp16/19 IMR90 cells. The images show the TUJ1- and MAP2- positive iN cells from shp16, shp19 and shp16/19 IMR90 fibroblasts 3 weeks after induction. Scale bar, 10 μm. ( d and e ) Quantitative analysis of iN cells from IMR90 cells with or without expressing shp16, shp19 or empty vector after induction. Kinetic analysis of iN purity was counted by morphology, TUJ1- (early stage, before one week induction) and MAP2-positive (late stage, after 1 week induction) staining, and the numbers represent the percentage of iN cells at the time point of quantification ( d ). Neuronal yield was determined as the percentage of MAP2+ cells in relation to the initial number of plated fibroblasts at 3 week after induction ( e ). Quantitative data were mean±s.e.m. from at least three independent experiments. 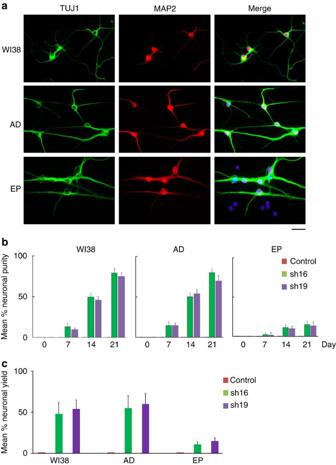Figure 2: iN cells from WI38, adult dermal fibroblasts (AD) and epithelia cells (EP) with expression of shp16. (a) shp16 iN cells 3 weeks after induction were positive stainings of MAP2 and TUJ1. Scale bar, 10 μm. (bandc) Quantitative analysis of iN cells from WI38, AD fibroblasts and EP cells with expression of sh16, sh19 or control empty vector. Kinetic analysis of iN purity was counted by TUJ1- and MAP2-positive staining (b). iN yield was determined at 3 weeks after induction (c). Quantitative method of iN purity and yield is the same as that inFig. 1. Quantitative data were mean±s.e.m. from three biologically independent experiments. Full size image Figure 2: iN cells from WI38, adult dermal fibroblasts (AD) and epithelia cells (EP) with expression of shp16. ( a ) shp16 iN cells 3 weeks after induction were positive stainings of MAP2 and TUJ1. Scale bar, 10 μm. ( b and c ) Quantitative analysis of iN cells from WI38, AD fibroblasts and EP cells with expression of sh16, sh19 or control empty vector. Kinetic analysis of iN purity was counted by TUJ1- and MAP2-positive staining ( b ). iN yield was determined at 3 weeks after induction ( c ). Quantitative method of iN purity and yield is the same as that in Fig. 1 . Quantitative data were mean±s.e.m. from three biologically independent experiments. Full size image So far, we identified iN cells based on their morphology and positive staining of several neuronal markers. Next, we further characterized the functional aspects of iN cells induced by shp16–shp19 from IMR90 cells. We found that ~75% of iN cells induced by depletion of p16–p19 showed synapsin-positive puncta that label the vesicles in the presynaptic nerve terminal ( Fig. 3a,b ). iN cells were positive in the immunostaining of vesicular glutamate transporter 1 (vGluT1, glutamatergic neuron marker) and GABA (GABAergic neuron marker), suggesting that iN cells could be either excitatory or inhibitory. Positive stainings of TBR1 and LHX6 in iN cells indicate that iN cells have the similar identities to forebrain neurons ( Fig. 3a,b ). They were negative in the immunostaining of peripherin (peripheral neuron marker) and tyrosine hydroxylase (dopaminergic neuron marker). 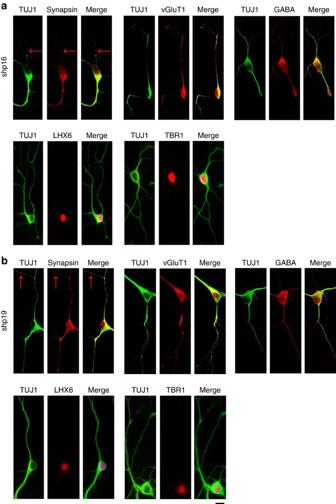Figure 3:p16andp19shRNAs directly convert human fibroblasts into functional neurons. (aandb) Expression of TUJ1, Synapsin, vGluT1, GABA, TBR1 and LHX6 in iN cells from shp16 (a) and shp19 (b) IMR90 fibroblasts 3 weeks after induction. Scale bar, 10 μm. Figure 3: p16 and p19 shRNAs directly convert human fibroblasts into functional neurons. ( a and b ) Expression of TUJ1, Synapsin, vGluT1, GABA, TBR1 and LHX6 in iN cells from shp16 ( a ) and shp19 ( b ) IMR90 fibroblasts 3 weeks after induction. Scale bar, 10 μm. Full size image To determine whether iN cells generate action potentials and neurotransmitter-induced currents, the basic functions of neurons, we cultured shp19 transfected IMR90 cells (7 days after induction) with a monolayer culture of primary rat neurons, which might provide a better environment for maturation [4] , [6] . iN cells were identified by green fluorescent protein fluorescence ( Supplementary Fig. 2 ). Two to three weeks after the co-culture, whole-cell voltage-clamp recordings of iN cells showed that 71% of iN cells exhibited inward fast activating and inactivating sodium currents and outward potassium currents during a ramp depolarization ( Fig. 4a , n =31). This was also confirmed by applying a series of voltage steps to evoke inward sodium currents and outward potassium currents ( Fig. 4b , 71%, n =31). Fast inward currents were blocked by application of tetrodotoxin, confirming that these inward currents were voltage-dependent sodium currents ( Fig. 4c , n =6). Moreover, single action potential or multiple action potential firings with an amplitude of 99.6±0.7 mV and width of 1.88±0.06 ms were detected using whole-cell patch clamp recording in shp19 induced neurons (3–4 weeks after induction; Fig. 4d , 71%, n =31). The induced neurons that could fire action potentials also responded to exogenous application of L-glutamate ( Fig. 4e , 89%, n =9) and GABA ( Fig. 4f , 70%, n =10), indicating the presence of functional glutamatergic and GABAergic postsynaptic terminals [22] . Even more importantly, miniature excitatory postsynaptic currents were recorded from induced neurons without co-culture, suggesting that iN cells can form functional synapses by themselves ( Fig. 4g ). We also obtained similar results from shp16 iN cells. These data indicate that iN cells induced by shp16 or shp19 are functional neurons. 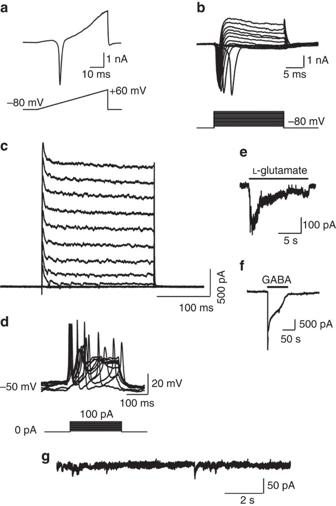Figure 4: Electrophysiological characterization ofshp19iNs from IMR90 fibroblasts. (a) Representative traces of membrane currents recorded with a ramp protocol (lower panel, a voltage ramp from −80 mV to +60 mV over 500 ms). Fast activating Na+ current was prominent. (b) Representative current traces (upper panel) recorded in voltage-clamp mode. Cells were depolarized by voltage steps from −80 to +60 mV in 10-mV increments (Δ10 mV, upper panel). The lower panel shows the current–voltage (I–V) relationship for sodium current. (c) Inward currents are tetrodotoxin-sensitive voltage-dependent sodium currents. (d) Traces of evoked action potentials in current-clamp mode. Step currents were injected from 0–100 pA in 10 pA increments. (eandf) Local application of either 15 mML-glutamate (e), or 15 mM GABA (f) elicited current responses. (g) miniature excitatory postsynaptic currents were recorded in voltage-clamp mode from shp19 iN cells without co-culture. Figure 4: Electrophysiological characterization of shp19 iNs from IMR90 fibroblasts. ( a ) Representative traces of membrane currents recorded with a ramp protocol (lower panel, a voltage ramp from −80 mV to +60 mV over 500 ms). Fast activating Na+ current was prominent. ( b ) Representative current traces (upper panel) recorded in voltage-clamp mode. Cells were depolarized by voltage steps from −80 to +60 mV in 10-mV increments (Δ10 mV, upper panel). The lower panel shows the current–voltage (I–V) relationship for sodium current. ( c ) Inward currents are tetrodotoxin-sensitive voltage-dependent sodium currents. ( d ) Traces of evoked action potentials in current-clamp mode. Step currents were injected from 0–100 pA in 10 pA increments. ( e and f ) Local application of either 15 mM L -glutamate ( e ), or 15 mM GABA ( f ) elicited current responses. ( g ) miniature excitatory postsynaptic currents were recorded in voltage-clamp mode from shp19 iN cells without co-culture. Full size image Senescence is a crucial step for neuron conversion Upregulation of p16 or p19, as well as activation of p53, induces cellular senescence [17] , [18] , [19] , [20] , [21] . When we repeated similar experiments in late stage IMR90 cells (population doublings PD 55), expression of shp16 or shp19 induced conversion at efficiency of ~10–15% after induction three weeks. The efficiency of conversion was in general much lower than that observed in early stage IMR90 cells, likely because the expression of p16 , p19 and p53 is progressively upregulated in late passage cells ( Fig. 5a ). A recent study showed that miR9-124+Ascl1/Neurod2/Mytl1 induced fibroblast–neuron conversion [7] . Consistently, expression of the set of miRNAs and transcription factors in IMR90 cells induced neuron conversion in IMR90 cells ( Supplementary Fig. 3 ). In parallel, p16 and p19 mRNA in fibroblasts and skin was significantly higher than the corresponding iN cells and cortex ( Fig. 5b ). These results raised a possibility that these genes might suppress fibroblast conversion to neurons, supporting that senescence is a crucial step for neuron conversion. To confirm whether the senescence process is involved in neuron conversion, we overexpressed wild-type p53 in IMR90 cells expressing shp16, shp19 or shp53 (3′UTR region). Expression of p53 essentially abolished fibroblast–neuron conversion throughout the 4 weeks we monitored ( Fig. 5c–e ), suggesting that p53 blocks the p16 and p19 pathway, consistent with previous reports that p16–p19 regulate p53 in cellular senescence [18] , [19] , [20] , [21] . 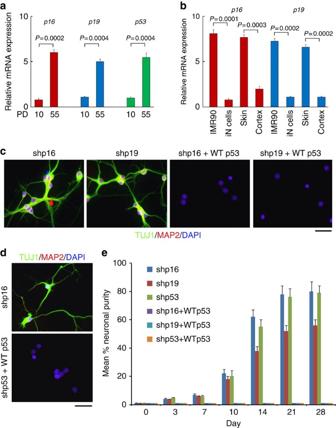Figure 5: Overcoming senescence induces iN conversion. (a) mRNA level ofp16, p19andp53in young and old IMR90 cells. mRNA expression levels of indicated genes were determined by quantitative reverse trancriptase–PCR in population doublings, PD10 and PD55 IMR90 cells. (b) mRNA expression ofp16andp19in different human cells and tissues (n=3) detected by quantitative reverse trancriptase-PCR. iN cells were from IMR90 cells expressing miRNA9-124+Ascl1/Myt1l/Neurod2. (candd) Wild-type p53 blocks conversion of IMR90 cells into iN cells induced by shp16, shp19 or shp53. Lentiviral wild-type p53 was expressed in IMR90 cells with expression of shp16, shp19 or shp53 (3′ UTR region). The images show the morphology of iN cells 4 weeks after induction. (e) Quantitative data represent mean % iN purity from shp16, shp19 and shp53 plus wild-type p53, respectively. After induction at the indicated time points, iN cells were identified by morphology, TUJ1 and MAP2-positive staining (see method inFig.1). Scale bar, 10 μm. (a,bande) Quantitative data are mean ±s.e.m. from three independent experiments. TheP-values are based on Student’st-test. Figure 5: Overcoming senescence induces iN conversion. ( a ) mRNA level of p16, p19 and p53 in young and old IMR90 cells. mRNA expression levels of indicated genes were determined by quantitative reverse trancriptase–PCR in population doublings, PD10 and PD55 IMR90 cells. ( b ) mRNA expression of p16 and p19 in different human cells and tissues ( n =3) detected by quantitative reverse trancriptase-PCR. iN cells were from IMR90 cells expressing miRNA9-124+Ascl1/Myt1l/Neurod2. ( c and d ) Wild-type p53 blocks conversion of IMR90 cells into iN cells induced by shp16, shp19 or shp53. Lentiviral wild-type p53 was expressed in IMR90 cells with expression of shp16, shp19 or shp53 (3′ UTR region). The images show the morphology of iN cells 4 weeks after induction. ( e ) Quantitative data represent mean % iN purity from shp16, shp19 and shp53 plus wild-type p53, respectively. After induction at the indicated time points, iN cells were identified by morphology, TUJ1 and MAP2-positive staining (see method in Fig.1 ). Scale bar, 10 μm. ( a , b and e ) Quantitative data are mean ±s.e.m. from three independent experiments. The P -values are based on Student’s t -test. Full size image hTERT eliminates barriers in fibroblast–neuron conversion To further confirm that the senescence pathway is involved in neuron induction from fibroblasts, we tested the activation of telomerase, which is a key mechanism by which cells escape senescence and become immortalized. Overexpression of hTERT, a telomerase enzymatic component, immortalizes primary fibroblasts. IMR90 cells are able to grow about 58 PDs before becoming senescent cells in normal culture condition (ATCC and Supplementary Fig. 4a ). We expressed hTERT in IMR90 cells ( Fig. 6a ) and found that these cells did have extended lifespan: they grew until 100 PDs ( Supplementary Fig. 4b ) and showed SA-β-Gal (a senescence marker) negative staining ( Fig. 6b ), indicating that the cells are immortalized. Next, we cultured hTERT IMR90 cells (PD 60) in neuronal induction medium and observed that 70–80% cells showed typical neuronal cell morphology in 5–7 days with TUJ1 and MAP2-positive staining ( Fig. 6c ). These induced neurons have functional voltage-dependent sodium currents and potassium currents, and can fire multiple action potentials ( Fig. 6d,e ). To confirm the effect of hTERT, we expressed hTERT in another normal human fibroblast cell line (WI38), cultured it in neuronal induction medium and observed that most of hTERT WI38 cells (~80%) became iN cells, similar to IMR90 cells ( Fig. 6f ). These data strongly support that overcoming replicative senescence may be critical during conversion of fibroblasts into neurons. 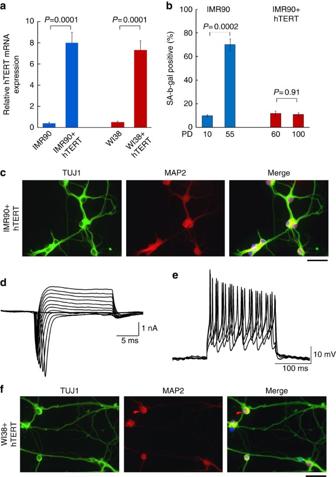Figure 6: Expression of hTERT induces fibroblasts into neurons. (a) Expression of hTERT in IMR90 and WI38 cells. IMR90 and WI38 fibroblasts were transduced with hTERT. Quantitative reverse trancriptase–PCR results show mRNA level ofhTERTin IMR90 and WI38 cells. TheP-values are based on Student’st-test. (b) Expression of SA-β-Gal in IMR90 and hTERT IMR90 cells. IMR90 control and hTERT cells were examined for SA-β-Gal activity at indicated population doublings. TheP-values are based on Student’st-test. (c) The images show the TUJ1- and MAP2- positive iN cells from hTERT IMR90 fibroblasts 1 week after induction. Scale bar, 10 μm. (d) Representative current traces recorded in voltage-clamp mode from hTERT IMR90 fibroblasts. Cells were depolarized by voltage steps from −80 to +60 mV in 10-mV increments (Δ10 mV). (e) Traces of evoked action potentials in current-clamp mode from hTERT IMR90 fibroblasts. Step currents were injected from 0–100 pA in 10-pA increments. (f) The images show the TUJ1- and MAP2- positive iN cells from hTERT WI38 fibroblasts 1 week after induction. Scale bar, 10 μm. Figure 6: Expression of hTERT induces fibroblasts into neurons. ( a ) Expression of hTERT in IMR90 and WI38 cells. IMR90 and WI38 fibroblasts were transduced with hTERT. Quantitative reverse trancriptase–PCR results show mRNA level of hTERT in IMR90 and WI38 cells. The P -values are based on Student’s t -test. ( b ) Expression of SA-β-Gal in IMR90 and hTERT IMR90 cells. IMR90 control and hTERT cells were examined for SA-β-Gal activity at indicated population doublings. The P -values are based on Student’s t -test. ( c ) The images show the TUJ1- and MAP2- positive iN cells from hTERT IMR90 fibroblasts 1 week after induction. Scale bar, 10 μm. ( d ) Representative current traces recorded in voltage-clamp mode from hTERT IMR90 fibroblasts. Cells were depolarized by voltage steps from −80 to +60 mV in 10-mV increments (Δ10 mV). ( e ) Traces of evoked action potentials in current-clamp mode from hTERT IMR90 fibroblasts. Step currents were injected from 0–100 pA in 10-pA increments. ( f ) The images show the TUJ1- and MAP2- positive iN cells from hTERT WI38 fibroblasts 1 week after induction. Scale bar, 10 μm. Full size image Genome-wide transcriptional profiling of induced neurons To analyse the similarities between iN cells and parental fibroblasts, we generated comparative global gene expression data by microarray analysis. Microarray data was quantile normalized and filtered based on the average signal, and differently expressed genes were selected for further analysis. Hierarchical cluster analysis revealed a significant difference between iN cells and their parental IMR90 cells ( Fig. 7a,b ). Although there are subtle differences in the global gene expression profiles of the iN cells tested (shp16 and hTERT), all of them are clearly distinct from both parental IMR90 and shp16 and hTERT IMR90 fibroblasts. In contrast, shp16 and hTERT IMR90 fibroblasts are similar to the parental IMR90 cells. The clustering analysis of global gene expression revealed that iN cells by miR9-124+Ascl1/Neurod2/Mytl1 are particularly similar to all of the iN cells by shp16 and hTERT ( Fig. 7a,b ), indicating that iN cells generated by different methods show similarity of gene expression profiling. By analysis of the threefold-changed genes of the microarray data, all iN cells showed the general degree of gene expression overlap ( Fig. 7c ). Using the Ontology data base for enrichment analysis, we found that the key signalling pathways involved in neuron differentiation were significantly changed in iN cells, compared with those in parental fibroblasts ( Fig. 7d ). These findings indicate that the genetic transdifferentiation erased the majority of the evident expression hallmarks of the cell of origin, whereas specifically inducing the neuronal phenotype. 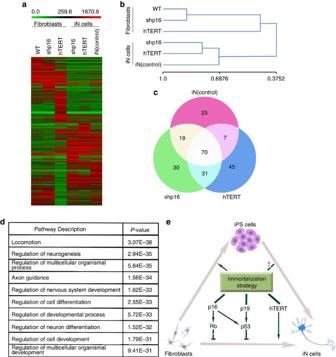Figure 7: Global gene expression profiling of iN cells. (a) Heat-map of genes differentially expressed in global RNA-microarray analysis performed on IMR90s (WT), IMR90 fibroblasts (expressing shp16, shp53 or hTERT) and iN cells (expression shp16, shp53 or hTERT and positive control (miRNA9-124+Ascl1/Myt1l/Neurod2)). (b) Hierarchical clustering. The numbers generated by MeV software represent the correlation among different samples. The bigger number represents the more similarity of the expression profiles among samples. (c) General degree of overlapping expression among the three cell populations analysed. To pick threefold-changed genes of the microarray data, 40–55% of genes (70 genes) from three iN groups showed the general degree of gene expression overlap. (d) Alterations of relevant pathways from Ontology data base in iN cells (shp16, shp53 and hTERT). (e) Schematic drawing of a proposed model for effects of immortalization on fibroblast–neuron conversion. Figure 7: Global gene expression profiling of iN cells. ( a ) Heat-map of genes differentially expressed in global RNA-microarray analysis performed on IMR90s (WT), IMR90 fibroblasts (expressing shp16, shp53 or hTERT) and iN cells (expression shp16, shp53 or hTERT and positive control (miRNA9-124+Ascl1/Myt1l/Neurod2)). ( b ) Hierarchical clustering. The numbers generated by MeV software represent the correlation among different samples. The bigger number represents the more similarity of the expression profiles among samples. ( c ) General degree of overlapping expression among the three cell populations analysed. To pick threefold-changed genes of the microarray data, 40–55% of genes (70 genes) from three iN groups showed the general degree of gene expression overlap. ( d ) Alterations of relevant pathways from Ontology data base in iN cells (shp16, shp53 and hTERT). ( e ) Schematic drawing of a proposed model for effects of immortalization on fibroblast–neuron conversion. Full size image Our results show that cellular senescence is a key step in the direct conversion of human fibroblasts into functional neurons ( Fig. 7e ). By genetically manipulating the senescence process by inhibition of Ink4/Arf or overexpression of hTERT, we provided a new method for converting fibroblasts into neural cells in only 1–2 weeks. The present work may improve the understanding of the mechanisms involved in cell transdifferentiation and reprogramming, particularly about the role of senescence. Direct lineage conversions between very distantly related cell types might involve two main steps: (1) reprogramming of prior donor cells, which might not pass through a pluripotent state; (2) subsequent redifferentiation into a complete and functional lineage. Our finding that overcoming senescence causes conversion of fibroblasts to neurons suggests that senescence may enhance both steps, consistent with the previous reports showing effects of the senescence pathway on reprogramming [15] , [23] , [24] . The ability to convert somatic cells into disease-relevant cell types through cellular reprogramming has opened new doors for basic research and regenerative medicine [1] . In the past, there were no reliable methods for converting non-neural somatic cells into neural cells. Takahashi et al. [1] demonstrated that defined factors could drive skin-derived fibroblasts to a pluripotent state that could be further differentiated into the desired cell type. However, robust differentiation into specific lineages remains a stumbling block. Low efficiencies and week-to-month-long protocols often give rise to mixed cultures requiring a second purification step. These iPS cells can also generate tumours after transplantation [25] , [26] , [27] , [28] , [29] . The field of direct somatic lineage conversion has already attracted much attention. Recently, Wernig’s group demonstrated that a set of neural factors can convert fibroblasts into neurons [4] , [6] . Several laboratories have used various neural factors and microRNAs to generate fibroblast–neuron conversion [7] , [13] , [30] , [31] . Furthermore, recent studies have reduced the numbers of transcription factors required for neuronal transdifferentiation by including small molecules to promote neuronal phenotypes [32] , [33] . We report here that inhibition of Ink4/Arf or overexpression of hTERT induces fibroblast–neuron conversion without introduction of any transcription factors. Global gene expression analysis reveals that the gene profiling in iN cells is significantly changed, compared with that in the parental fibroblasts, supporting the notion that Ink4/Arf and hTERT may act as a ‘master switch’ to coordinate a set of defined factors in regulating cell reprogramming. Consistent with this view, overcoming senescence enhances both iPS reprogramming and neural conversion, implicating a general mechanism of reprogramming where overcoming senescence may generate and develop complete and functional lineages. One hypothesis is that overcoming senescence prevents loss of proliferative potential in cell cycle-arrested cells and that it can therefore transform irreversible arrest into a reversible condition. When the cell cycle is arrested by neural induction medium (for fibroblast–neuron conversion) or reprogramming factors (for iPS cell formation), in the absence of Ink/Arf, the cells remain quiescent but not senescent because they retain the capacity to resume proliferation. Under defined conditions, the cells are reprogrammed into progenitors and sequentially redifferentiated into neural lineages or continue to reprogram into iPS cells. Therefore, the signalling molecules (for example, BDNF, dbcAMP) in the defined induction culture medium also play important roles in the transdifferentiation process, as these are likely to be essential for promoting neurogenesis, facilitated by reduction in Ink4 and Arf expression. In addition, these signalling molecules might promote neuronal survival and maturation [7] . Direct neuron conversion by introduction of defined factors might have significant implications for understanding critical processes for neuronal development, in vitro disease modelling and cell replacement therapies, although generally with low percentages and very slow time course of conversion [30] , [31] , [34] . Delineating the molecular mechanism behind neuron conversion can add logic to the method. Our findings may have wide-spread impact on our understanding and development of neuron replacement therapy. Although the link between p16–p19 and tumorigenicity makes using the iN cells lacking p16–p19 impractical, treating cells during conversion with reversible compounds to promote immortalization transiently is feasible. In the future, testing compounds that block senescence for neuron conversion may be a novel approach for maximizing the generation of “safe” neurons for clinical applications, including for old people who may suffer more neurological disorders. We believe that senescence will be a key process to target in pursuit of finding more efficient strategies for generating iN cells. Cell culture Human fibroblasts from ATCC (IMR90, a line of lung-derived fibroblasts from 16 weeks gestation fetus; WI38, a line of lung fibroblasts from 3 months gestation fetus and adult dermal fibroblasts derived from a 46-year old healthy male donor) were routinely cultured in 60 mm dish (MidSci) in Dulbecco’s modified Eagle medium (Hyclone) containing 10% fetal bovine serum (Sigma), non-essential amino acids (Invitrogen) and penicillin/streptomycin (Invitrogen) at 37 °C in 5% CO 2 . Primary normal human bronchial/tracheal epithelial cells (from a 34-year-old female donor) were from ATCC (PCS-300-010). Neural cell conversion For neuronal conversion, modified fibroblasts were plated in human esophageal fibroblast medium at a density of 3.0 × 10 4 cells cm −2 on microscope glass coverslips coated with Matrigel (BD) in 35 mm dish. Four days after infection, the media was changed to defined neuronal induction media including Neuronal Media (ScienCell) plus 0.5 mM Dibutyryl cyclic-AMP sodium salt (dbcAMP, Sigma), 20 ng ml −1 basic Fibroblast Growth Factor (ScienCell) with medium changes every 4 days. We also added 10 ng ml −1 human brain-derived neurotrophic factor (BDNF) and Neurotrophin-3 (NT3; both from PROSPEC) after 2 weeks to the medium to enhance induced cell survival. Quantitative of mean % iN purity is counted by morphology, TUJ1- (early stage, before one week induction) and MAP2-positive (late stage, after one week induction) staining, and the numbers represent the percentage of iN cells at the time point of quantification. Mean % neuronal yield is determined as the percentage of MAP2+ cells in relation to the initial number of plated fibroblasts at 3 week after induction. Cortical neuron culture and co-culture with iNs Primary cortical neurons were isolated from P0 rat. Cortices were dissected and dissociated by trypsin digestion (0.25% Trypsin, 137 mM NaCl, 5 mM KCl, 7 mM Na 2 HPO 4 , 25 mM HEPES) and plated on poly- D -lysine coated glass coverslips. The neurons were maintained in growth media consisting of MEM supplemented with B27, glutamine (all from Invitrogen), glucose, transferrin (Calbiochem), fetal bovine serum and Ara-C (both from Sigma) for a week before co-culture with iNs. iNs were induced for 7 days by Induction Medium (Neuronal medium (ScienCell), 20 ng ml −1 human basic Fibroblast Growth Factor, 1 mM Valproic acid) and dissociated by trypsin digestion (0.05% Trypsin). Then iN cells were seeded onto cortical neurons bed and maintained in Mature Medium (Induction Medium with 0.5 mM dbcAMP, 10 ng ml −1 BDNF, 10 ng ml −1 NT3). Mature Medium was replaced every 2 days. Viral preparation and western blot cDNA of neural transcription factors Ascl1 , Brn2 , NeuroD2 , Myt1l and miR9-124 were gifts from Andrew S. Yoo. The following shRNAs (Sigma) were used: sh p16 at cDNA (accession number NM_058197), positions 401-421(5′-GCGCTGCCCAACGCACCGAAT-3′); sh p19 at cDNA, positions 332-546(5′-GCTGATCTTCTCCAAGAGGAA-3′); sh p16/19 at 3′UTR, positions 1335-1355 (5′-CGCACATTCATGTGGGCATTT-3′); Western blotting analyses were performed to check the knock down efficiency. Immunofluorescence Immunofluorescence staining was performed as following. 5 × 10 4 modified human fibroblasts were planted on Matrigel-coated glass coverslips the day before induction. Ten to 28 days after viral infection, cells were fixed for 20 min at room temperature in 4% paraformaldehyde in PBS, permeabilized for 30 min in PBS containing 0.2% Triton X-100 and 10% normal goat serum (NGS) and incubated overnight at 4 °C in PBS containing 10% NGS and primary antibodies. Then cells were washed three times with PBS and incubated for 2 h at room temperature with anti-rabbit or anti-mouse secondary antibodies Alexa Fluor-488 or Alexa Fluor-594 (1:500, Invitrogen). The images were acquired by immunofluorescence microscope or Zeiss LSM 510 META confocol microscope with × 40, 1.3 numerical aperture oil-immersion objective. The following antibodies were used for the immunofluorescence studies: rabbit anti-MAP2 (Sigma-Aldrich, 1:200), mouse anti-Tuj1 (R&D Systems, 1:100), mouse anti-synaptotagmin 1 (Synaptic Systems, 1:100), rabbit anti-synapsin 1(Cell Signaling, 1:200), Rabbit anti-synapsin (1:1,000, Millipore), Guinea pig anti-vGluT1 (1:5,000, Millipore), rabbit anti-GABA (1: 3,000, Sigma), mouse anti-peripherin (1:100, Millipore), mouse anti-tyrosine hydroxylase (1:8,000, Sigma), mouse anti-TUJ-1 (1:1,000, Covance) and rabbit anti-TUJ-1 (1:2,000, Covance). qRT-PCR Total RNA was extracted using Trizol isolation system (Invitrogen) according to the manufacturer’s instructions. Total RNA was treated with DNase I (Qiagen) to prevent DNA contamination. Two micrograms of RNA were reverse transcribed using the Transcriptor High Fidelity cDNA Synthesis Kit (Roche). Reverse transcription and real-time PCR were performed as a standard procedure. Electrophysiology Coverslips with iNs were placed in the recording chamber mounted on an Olympus 1 × 81 microscope. All electrophysiology recordings were recorded at room temperature (22–25 °C) via whole-cell recording with a patch electrode. Signals were amplified using Heka EPC-10 amplifier and filtered at 2 KHz via a Bessel low-pass filter. Data were samples using Puls8.8 software, and analysed using Igor6.04. For recording voltage-gated currents and action potentials, patch electrodes were filled with solution (in mM): 130 K-gluconate, 10 KCl, 10 HEPES, 0.5 EGTA, 4 MgATP, 0.3 Na2GTP, 10 P-Creatin, pH adjusted by KOH to 7.2, osmolarity measured at 310 mOsm. The composition of the external solution used for recording was as follows (in mM): 105 NaCl, 25 NaHCO3, 3 Myo-Inositol, 2 Na-Pyruvate, 2.5 KCl, 1.25 NaH2PO4, 25 Glucose, 2 CaCl2, 1.5 MgCl2, pH adjusted by NaOH to 7.4, osmolarity measured at 300 mOsm. To isolate voltage-dependent sodium currents, 1 μM tetrodotoxin was added to the external solution. To monitor voltage-gated currents, we applied step potentials ranging from −60 mV to +60 mV for 20 ms. To monitor action potentials, we applied step currents ranged from 10–100 pA for 200 ms. L-Glutamate and GABA were prepared in bath solution and applied by an electrode placed 50–70 μm from the cells. External solutions changes were achieved rapidly, within 100 ms. Microarray analysis RNA was prepared as described in quantitative reverse transcriptase–PCR section. Microarray analysis was performed at the Washington University Genome Center. Briefly, Illumina HumanHT-12 v4 Expression BeadChip was used and samples were labelled by biotin. The Direct Hybridization Assay was performed and the data were scanned on the BeadArray Reader. Scanned images were quantitated by Illumina Beadscan, v3. Quantitative data was imported into Illumina GenomeStudio software and normalized by Illumina’s quantile method. The quantile-normalized background-subtracted data were calculated in excel. The data were filtered based on the average signal, and set the baseline as 50 so that only the genes of which average signal >50 could be used for further analysis. To each gene, maximum and minimum signal values were selected, and then divided between them. Only the genes of the division value >3 were selected and considered as differently expressed. All of the differently expressed genes were clustered by using MeV software. To determine the relationship between fibroblasts and iN cells, each iN sample was analysed respectively. The iN cells derived from shp16 and hTERT were compared with fibroblasts and positive control iN cells derived from miR-9-124+Ascl1/NeuroD2/Myt1l. Data were filtered based on average signal and baseline was set as 10 to increase the sensitivity. Differently expressed genes between shp16, hTERT and iN (positive control) samples and wild-type IMR90 cells were selected by threefolds changed as threshold. To examine the potential neuron differentiation pathways relevant to the immortalization, all neuron differentiation genes from Gene Ontology Website ( http://www.geneontology.org/ , GO: 0030182; total 1,003 genes) were compared with the microarray data. For gene enrichment analysis, we used web-based Gorilla programme ( http://cbl-gorilla.cs.technion.ac.il/ ). The total 101 genes were selected from overlapping between the p16/hTERT groups and all neuron differentiation genes from Ontology. How to cite this article: Sun, C.-k. et al. Senescence impairs direct conversion of human somatic cells to neurons. Nat. Commun. 5:4112 doi: 10.1038/ncomms5112 (2014).